Interferon-γ-producing immature myeloid cells confer protection against severe invasive group AStreptococcusinfections Cytokine-activated neutrophils are known to be essential for protection against group A Streptococcus infections. However, during severe invasive group A Streptococcus infections that are accompanied by neutropenia, it remains unclear which factors are protective against such infections, and which cell population is the source of them. Here we show that mice infected with severe invasive group A Streptococcus isolates, but not with non-invasive group A Streptococcus isolates, exhibit high concentrations of plasma interferon-γ during the early stage of infection. Interferon-γ is necessary to protect mice, and is produced by a novel population of granulocyte–macrophage colony-stimulating factor-dependent immature myeloid cells with ring-shaped nuclei. These interferon-γ-producing immature myeloid cells express monocyte and granulocyte markers, and also produce nitric oxide. The adoptive transfer of interferon-γ-producing immature myeloid cells ameliorates infection in wild-type and interferon-γ-deficient mice. Our results indicate that interferon-γ-producing immature myeloid cells have a protective role during the early stage of severe invasive group A Streptococcus infections. Streptococcus pyogenes (group A Streptococcus ; GAS) is one of the most common human pathogens. It causes a wide variety of infections, ranging from uncomplicated pharyngitis and skin infections to severe and even life-threatening manifestations such as streptococcal toxic shock syndrome (STSS) and necrotizing fasciitis. The mortality rates for STSS and necrotizing fasciitis are high (30–70%), even following prompt antibiotic therapy and debridement [1] , [2] , [3] , [4] . It is widely believed that myeloid cells including polymorphonuclear leukocytes (PMNs) have a central role in survival from GAS infections, and interferon (IFN)-γ is essential to full activation and proper function of PMNs. Notably, IFN-γ at the infection site is thought to be critical for protection; however, its increased systemic levels seem to be detrimental to survival after GAS infections [5] . Therefore, the appropriate regulation of cytokine-producing cells may be critical for survival and host defense against severe invasive GAS infections. Myeloid cells with ring-shaped nuclei (ring cells) are present in the peripheral blood of patients with myeloproliferative diseases, but only rarely in healthy control subjects [6] , [7] . Ring cells are usually referred to as PMNs. However, not only Gr-1 high PMN-like ring cells, but also Gr-1 low mononuclear cell-like ring cells are present in the bone marrow, peripheral blood, and inflammatory infiltrates of mice [8] . Morphologically, a part of myeloid-derived suppressor cells (MDSCs) has ring-shaped nuclei [9] , [10] . MDSCs are potent suppressors of T-cell immunity, and their presence is associated with a poor clinical outcome in cancer. They are divided into 2 subtypes according to morphology and surface markers: Ly-6G − Ly-6C high monocytic MDSCs and Ly-6G + Ly-6C low granulocytic MDSCs [11] , [12] . Recent studies have demonstrated the considerable suppressive potential of MDSCs on T-cell immunity in autoimmune diseases, and also in chronic infections with intracellular pathogens, such as Salmonella typhimurium , Candida albicans , Trypanosoma cruzi , and Toxoplasma gondii [13] . However, the biological functions of ring cells in infectious diseases, and also the relationship between ring cells and MDSCs, remain largely unknown. In the present study, IFN-γ-producing immature myeloid cells with ring-shaped nuclei (γIMCs), which originated from bone marrow precursor-like cells (BMPCs), are shown to be functionally and phenotypically distinct from MDSCs. We demonstrate that γIMCs have a protective role against severe invasive GAS infections, and possibly compensate for neutropenia. Role of IFN-γ in severe invasive GAS infections To clarify the types of cytokines involved in severe invasive GAS infections, we first investigated the dynamics of cytokines in severe invasive and non-invasive GAS infections. As a model of disseminated infection in normally sterile sites, we intraperitonially (i.p.) infected GAS-susceptible C3H/HeN mice [14] , [15] , [16] , [17] with either severe invasive ( emm3 genotype rgg gene-mutated STSS strain, NIH34) or non-invasive ( emm3 genotype non-STSS (pharyngitis) strain, K33) GAS clinical isolates [18] , and measured the levels of plasma cytokines. We detected no significant amount of plasma cytokines within 24 h of infection. By contrast, in mice infected with severe invasive GAS isolates, but not with non-invasive GAS isolates, we detected high levels of plasma IFN-γ; moreover, the levels increased rapidly at 48 h post-infection ( Fig. 1a ). Other cytokines, such as IL-1α, IL-1β, IL-4, IL-5, IL-12 p70 and IL-17, were scarcely detected in the plasma of mice infected with either severe invasive or non-invasive isolates. By contrast, in mice infected with severe invasive GAS isolates, the levels of IL-2, IL-10, and TNF increased transiently at 36 h post-infection. 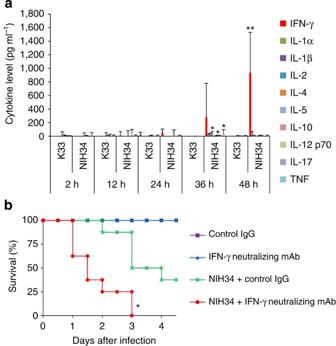Figure 1: IFN-γ is a host defense factor in mice infected with severe invasive GAS isolates. (a) C3H/HeN mice were i.p. inoculated withS. pyogenes(emm3genotype) clinical isolates (non-STSS, K33; STSS, NIH34; 3.0×107CFU per mouse), and plasma cytokine levels were determined by FlowCytomix. Data are expressed as mean±s.d. for at least 2 independent experiments, using a total of 6–10 mice for each group. The differences compared with K33-infected mice were statistically significant (*P<0.05, **P<0.01) as determined by Student'st-test. (b) C3H/HeN mice were i.p. inoculated with NIH34 (3.0×107CFU per mouse) in the presence of an IFN-γ neutralizing mAb (clone R4-6A2) (1 mg per mouse) or control rat IgG (1 mg per mouse). Survival was observed for 4 days post-infection. Mortality differences compared with infected mice in the presence of control IgG were statistically significant (*P<0.05), as determined by a log-rank test. Survival curves were generated from two independent experiments, using a total of eight mice for each group. Figure 1: IFN-γ is a host defense factor in mice infected with severe invasive GAS isolates. ( a ) C3H/HeN mice were i.p. inoculated with S. pyogenes ( emm3 genotype) clinical isolates (non-STSS, K33; STSS, NIH34; 3.0×10 7 CFU per mouse), and plasma cytokine levels were determined by FlowCytomix. Data are expressed as mean±s.d. for at least 2 independent experiments, using a total of 6–10 mice for each group. The differences compared with K33-infected mice were statistically significant (* P <0.05, ** P <0.01) as determined by Student's t -test. ( b ) C3H/HeN mice were i.p. inoculated with NIH34 (3.0×10 7 CFU per mouse) in the presence of an IFN-γ neutralizing mAb (clone R4-6A2) (1 mg per mouse) or control rat IgG (1 mg per mouse). Survival was observed for 4 days post-infection. Mortality differences compared with infected mice in the presence of control IgG were statistically significant (* P <0.05), as determined by a log-rank test. Survival curves were generated from two independent experiments, using a total of eight mice for each group. Full size image Further, we evaluated whether IFN-γ is the host factor contributing to protection against severe invasive GAS infections, or to deterioration of STSS through an augmented inflammatory process. We i.p. administered mice with an anti-mouse IFN-γ neutralizing mAb (clone R4-6A2), on the day of infection with severe invasive GAS isolates. At 72 h post-infection, all of the mice administered with the IFN-γ neutralizing mAb died. By contrast, 50% of the mice treated with rat IgG as a control survived ( Fig. 1b ). These results are consistent with those of a previous study [5] , in which mice treated with a different IFN-γ neutralizing mAb (clone XMG1.2) and IFN-γ knockout ( Ifng −/− ) mice were more susceptible to lethal skin infection with the M-nontypeable GAS strain 64/14 than were control IgG-administered mice and wild-type mice, respectively. Thus, IFN-γ may act as a host defense factor against severe invasive GAS infections. A source of IFN-γ in severe invasive GAS infections It is widely believed that T cells are a main source of IFN-γ in severe invasive GAS infections [19] , [20] , [21] . To identify the IFN-γ-producing cell types in mice infected with severe invasive GAS isolates, we used an in vivo intracellular cytokine synthesis (ICS) assay [22] , [23] to assess splenic IFN-γ production at 48 h post-infection. Unexpectedly, we revealed that Gr-1 + CD11b + cells (but not TCR-β + TCR-γ/δ + , CD4 + , or CD8 + T cells, DX5 + NK/NKT cells, or CD11c + MHC-II + dendritic cells) were a source of splenic IFN-γ in superantigen-insensitive C57BL/6 mice [24] , [25] , and also in C3H/HeN mice ( Fig. 2a and b ). These Gr-1 + cells appeared in the spleen on day 1 post-infection, subsequently increased in number, and were the major source of IFN-γ throughout infection ( Supplementary Fig. S1 ). By contrast, TCR-β + T cells and DX5 + or NK1.1 + NK cells, which are regarded as the sources of IFN-γ in GAS infections [15] , [16] , [17] , produced small amounts of IFN-γ during the late stage (days 3–5 post-infection) of severe invasive GAS infections in C3H/HeN mice, but not in C57BL/6 mice. Notably, the accumulation of Gr-1 + cells led to the clearance of infection from the spleen. Additionally, the administration of monensin, which blocks intracellular cytokine transport, did not induce spontaneous splenic production of IFN-γ ( Fig. 2a and b ; Supplementary Fig. S1 ). 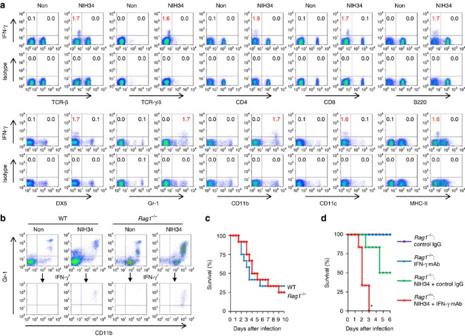Figure 2: CD11b+Gr-1+cells are the source of IFN-γ in severe invasive GAS infections. (a,b) C3H/HeN mice (a), C57BL per six mice (WT) (b), andRag1−/−mice (b) with or without i.p. infection of NIH34 (3.0×107CFU per mouse) for 42 h were i.v. injected with monensin. Six hours later, the mice were sacrificed and their splenocytes were immediately stained for the indicated markers, and analysed by ICS assay. (a) The numbers (%) in the plots represent the proportion of IFN-γ+subsets to total splenocytes. (b) Lower panels show the cells gated on the IFN-γ+population. Data are representative of three independent experiments. (c,d) WT andRag1−/−mice were i.p. inoculated with NIH34 (3.0×107CFU per mouse) in the absence (c) or presence (d) of an IFN-γ neutralizing mAb (clone R4-6A2) or control rat IgG (1 mg per mouse) as inFig. 1b. Survival (in days) was observed as indicated. Survival curves were generated from 2 independent experiments, using a total of 12 mice for each group. (d) Mortality differences compared with infected mice in the presence of control IgG were statistically significant (*P<0.05) as determined by a log-rank test. Figure 2: CD11b + Gr-1 + cells are the source of IFN-γ in severe invasive GAS infections. ( a , b ) C3H/HeN mice ( a ), C57BL per six mice (WT) ( b ), and Rag1 −/− mice ( b ) with or without i.p. infection of NIH34 (3.0×10 7 CFU per mouse) for 42 h were i.v. injected with monensin. Six hours later, the mice were sacrificed and their splenocytes were immediately stained for the indicated markers, and analysed by ICS assay. ( a ) The numbers (%) in the plots represent the proportion of IFN-γ + subsets to total splenocytes. ( b ) Lower panels show the cells gated on the IFN-γ + population. Data are representative of three independent experiments. ( c , d ) WT and Rag1 −/− mice were i.p. inoculated with NIH34 (3.0×10 7 CFU per mouse) in the absence ( c ) or presence ( d ) of an IFN-γ neutralizing mAb (clone R4-6A2) or control rat IgG (1 mg per mouse) as in Fig. 1b . Survival (in days) was observed as indicated. Survival curves were generated from 2 independent experiments, using a total of 12 mice for each group. ( d ) Mortality differences compared with infected mice in the presence of control IgG were statistically significant (* P <0.05) as determined by a log-rank test. Full size image To exclude the involvement of T cells in protection against severe invasive GAS infections, we investigated IFN-γ production in C57BL/6.RAG1 knockout ( Rag1 −/− ) mice, which have no mature B and T cells [26] . The ICS assay revealed that the cellular source of IFN-γ during severe invasive GAS infections was Gr-1 + CD11b + cells in Rag1 −/− mice, and also in C57BL/6 wild-type (WT) mice ( Fig. 2b ). We further examined the mortality of Rag1 −/− mice during severe invasive GAS infections. We observed no significant difference in mortality between Rag1 −/− and WT mice infected with severe invasive GAS isolates ( Fig. 2c ). Furthermore, similar to C3H/HeN mice ( Fig. 1b ), IFN-γ neutralizing mAb (clone R4-6A2)-treated Rag1 −/− mice were more susceptible to severe invasive GAS infections than were control IgG-administered Rag1 −/− mice ( Fig. 2d ). Our results indicate that mature B and T cells do not affect the mortality of infected mice, and that T cells have no protective effect during the early stage of severe invasive GAS infections. Characterization of the early source of IFN-γ Anti-Gr-1 mAb detects Ly-6C + monocytes and Ly-6G + PMNs. Therefore, to determine which subset of Gr-1 + CD11b + cells is responsible for IFN-γ production during severe invasive GAS infections, we investigated the surface phenotype of IFN-γ-producing cells isolated from the spleens of mice at 48 h post-infection. The ICS assay revealed that IFN-γ-producing cells had the phenotype of monocytes (F4/80 low CX3CR1 + ) and PMNs (Ly-6G + Ly-6C low ) ( Fig. 3 ). Additionally, they expressed no lymphoid (CD27, IL-7Rα) or granulocyte-lineage (CCR3, Siglec-F, c-Kit, IL-5Rα (H7)) markers, but exhibited particular profiles of CCR2 − CD31 + CD34 − CD38 + CD44 high CD49d + CD62L + CD69 + IL-5Rα (T21) high Siglec-H − ( Fig. 3 ; Supplementary Table S1 ). In this model, the most prominent GAS infection was present in the kidney [18] , [27] . In accordance with the bacterial burden in the peritoneal cavity, spleen and kidney, a higher proportion of IFN-γ-producing cells accumulated in the kidney of C3H/HeN mice, and also C57BL/6 mice i.p. infected with NIH34 ( Supplementary Fig. S2 ). By contrast, lower proportion of IFN-γ-producing cells existed at the sites of infection. A skin-infection model yielded similar results ( Supplementary Fig. S2 ). Furthermore, IFN-γ-producing cells were detected in the spleens from mice infected with various STSS strains [18] , [27] ( Supplementary Fig. S3 ). These cells were also detected in the peripheral blood and (in particularly high frequency) the bone marrow from NIH34-infected mice ( Fig. 4a–d ; Supplementary Fig. S4 ). Interestingly, Siglec-F + eosinophils (Eos) stained with IL-5Rα (H7) and IL-5Rα (T21), whereas IFN-γ-producing cells stained well with T21, but not with H7 ( Fig. 4e ), suggesting that IFN-γ-producing cells were phenotypically distinct from Eos. IFN-γ-producing cells were also phenotypically distinct from Ly-6C low CD31 − PMNs ( Fig. 4d ). Moreover, the number and proportion of PMNs were markedly reduced in the spleen, peripheral blood, and bone marrow at 48 h post-infection ( Fig. 4d and f ), as reported in human STSS cases [28] . 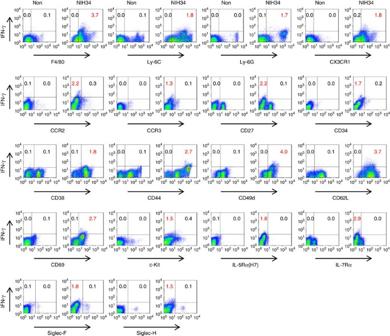Figure 3: IFN-γ-producing cells exhibit monocyte and PMN phenotypes in severe invasive GAS infections. C3H/HeN mice with or without i.p. infection of NIH34 (3.0×107CFU per mouse) for 42 h were i.v. injected with monensin. Six hours later, the mice were killed and their splenocytes were immediately stained for the indicated markers, and analysed by the ICS assay. The numbers (%) in the plots represent the proportion of IFN-γ+subsets to total splenocytes. These data are representative of three independent experiments. Figure 3: IFN-γ-producing cells exhibit monocyte and PMN phenotypes in severe invasive GAS infections. C3H/HeN mice with or without i.p. infection of NIH34 (3.0×10 7 CFU per mouse) for 42 h were i.v. injected with monensin. Six hours later, the mice were killed and their splenocytes were immediately stained for the indicated markers, and analysed by the ICS assay. The numbers (%) in the plots represent the proportion of IFN-γ + subsets to total splenocytes. These data are representative of three independent experiments. 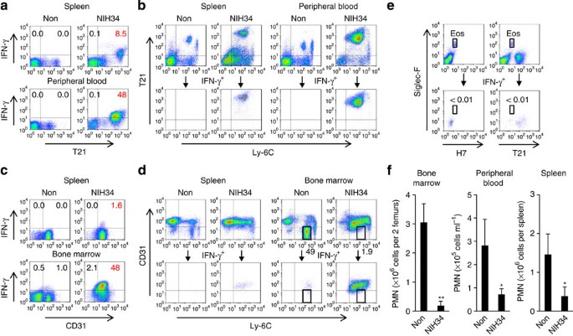Figure 4: IFN-γ-producing cells are detected in the peripheral blood and the bone marrow of GAS-infected mice. (a–d) Non-infected C3H/HeN mice or (a–e) mice i.p. infected with NIH34 (3.0×107CFU per mouse) for 42 h were i.v. injected with monensin. Six hours later, the mice were killed and their splenocytes (a–e), peripheral blood cells (a,b), and bone marrow cells (c,d) were immediately stained for the indicated markers, and analysed by ICS assay. (a,c) The numbers (%) in the plots represent the proportion of IFN-γ+subsets to total cells. (b,d,e) Lower panels show the cells gated on the IFN-γ+population. (d,e) Rectangle gates in the plot represent mature granulocytes (d) and Eos (e). The numbers (%) in the plots represent the proportion of mature granulocytes (d) or IFN-γ+Eos (e) to total cells. Data are representative of three independent experiments. (f) The numbers of PMNs in the bone marrow, peripheral blood, and spleen from non-infected or NIH34-infected mice at 48 h. Data are expressed as mean±s.d. (n=3). The differences compared with non-infected mice were statistically significant (*P<0.05, **P<0.01) as determined by Student'st-test. Full size image Figure 4: IFN-γ-producing cells are detected in the peripheral blood and the bone marrow of GAS-infected mice. ( a–d ) Non-infected C3H/HeN mice or ( a–e ) mice i.p. infected with NIH34 (3.0×10 7 CFU per mouse) for 42 h were i.v. injected with monensin. Six hours later, the mice were killed and their splenocytes ( a–e ), peripheral blood cells ( a , b ), and bone marrow cells ( c,d ) were immediately stained for the indicated markers, and analysed by ICS assay. ( a , c ) The numbers (%) in the plots represent the proportion of IFN-γ + subsets to total cells. ( b , d , e ) Lower panels show the cells gated on the IFN-γ + population. ( d , e ) Rectangle gates in the plot represent mature granulocytes ( d ) and Eos ( e ). The numbers (%) in the plots represent the proportion of mature granulocytes ( d ) or IFN-γ + Eos ( e ) to total cells. Data are representative of three independent experiments. ( f ) The numbers of PMNs in the bone marrow, peripheral blood, and spleen from non-infected or NIH34-infected mice at 48 h. Data are expressed as mean±s.d. ( n =3). The differences compared with non-infected mice were statistically significant (* P <0.05, ** P <0.01) as determined by Student's t -test. Full size image Immature myeloid cells as an early source of IFN-γ The IFN-γ-producing cells expressed the phenotypic markers of monocytes/macrophages (F4/80 and CX3CR1) and PMNs (Ly-6G). Therefore, we sorted CD11b + CD11c − F4/80 low Ly-6G + cells from the spleens of infected mice and morphologically analysed them with May-Grünwald-Giemsa staining. The IFN-γ-producing CD11b + CD11c − F4/80 low Ly-6G + splenocytes were IMCs, but not monocytes/macrophages or PMNs. These IFN-γ-producing IMCs were large cells containing ring-shaped, non-segmented nuclei, with a coarse chromatin pattern [6] , [7] , [8] ( Fig. 5a and b ). The sorted cells were contaminated with a small number of PMNs; however, immunohistochemical analyses showed that IMCs, but not PMNs, were the source of IFN-γ ( Fig. 5c ). The cells with ring-shaped nuclei were also observed in the peritoneum, kidney, and spleen from i.p. infection model, and in the skin from subcutaneous (s.c.) infection model, whereas such cells were not observed in the spleen and kidney from non-infected or non-invasive K33 strain-infected mice ( Fig. 5d and e ). To determine whether IFN-γ-producing IMCs (γIMCs) are committed to the granulocyte or monocyte lineage, we cultured sorted CD11b + CD11c − F4/80 low Ly-6G + γIMCs in vitro , in the presence of G-CSF, M-CSF, GM-CSF or IL-5. We observed that G-CSF, M-CSF and IL-5 failed to promote differentiation and survival ( Fig. 5f ). By contrast, in the presence of GM-CSF, differentiated γIMCs increased their expression of CD11c, F4/80, DX5 and Siglec-F ( Fig. 5g ) with the polymorphonuclear phenotype ( Fig. 5h ). Such granulocyte-like cells showed reduced ability to produce IFN-γ ( Fig. 5i ), and were phenotypically different from c-Kit low H7 + Siglec-F + bone marrow-derived Eos and CCR3 + H7 + Siglec-F + splenic Eos [29] ; ( Supplementary Fig. S5 ). These results suggest that γIMCs are committed to the granulocyte lineage, but do not exist in the steady state, and produce IFN-γ during a specific stage of differentiation. 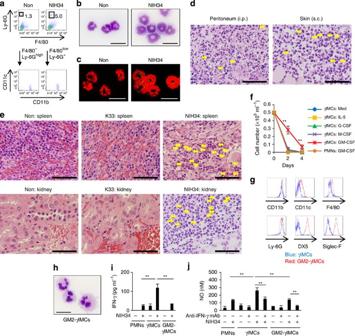Figure 5: γIMCs are the source of IFN-γ in severe invasive GAS infections. (a) CD11b+CD11c−F4/80−Ly-6GhighPMNs in splenocytes from non-infected C3H/HeN mice, or CD11b+CD11c−F4/80lowLy-6G+γIMCs in splenocytes from mice infected with NIH34, were isolated by FACS. (b,c) Cytospin preparations of each sorted cell type were visualized with May-Grünwald-Giemsa staining (b), whereas intracellular IFN-γ (green, IFN-γ; red, nuclei) was visualized with a confocal laser microscopy (c). Scale bars, 20 μm. (d,e) Paraffin-embedded sections of peritoneum, from mice i.p. infected with NIH34 and skin from mice subcutaneously (s.c.) infected with NIH34 for 48 h (d), and of spleen and kidney from mice i.p. infected with or without K33 or NIH34 for 48 h, (e) were visualized with hematoxylin and eosin staining. The yellow arrows indicate the cells with ring-shaped nuclei. Scale bars, 100 μm. (f) Sorted IMCs were cultured with control medium (Med), G-CSF (50 ng ml−1), M-CSF (10 ng ml−1), GM-CSF (10 ng ml−1), or IL-5 (10 ng ml−1) for 2–4 days, and their absolute numbers were counted on the indicated days. Data are expressed as the average (mean±s.d.) of triplicate wells (n=3). The differences compared with Med were statistically significant (**P<0.01) as determined by Student'st-test. (g) γIMCs (blue line) and GM-CSF (2 days)-cultured γIMCs (GM2-γIMCs: red line) were stained for the indicated markers. Data are representative of three independent experiments. (h) Cytospin preparations of GM2-γIMCs were visualized with May-Grünwald-Giemsa staining. Scale bars, 20 μm. (i,j) γIMCs and GM2-γIMCs were cultured with erythromycin-treated NIH34 (MOI 100) in the presence of control rat IgG or an IFN-γ neutralizing mAb (clone R4-6A2) for 24 h. The levels of IFN-γ (i) and NO2−(j) in the culture supernatants were measured by ELISA and Griess reagent system, respectively. The average (mean±s.d.) of triplicate wells is shown. Statistical significance (**P<0.01) was determined by ANOVA. Figure 5: γIMCs are the source of IFN-γ in severe invasive GAS infections. ( a ) CD11b + CD11c − F4/80 − Ly-6G high PMNs in splenocytes from non-infected C3H/HeN mice, or CD11b + CD11c − F4/80 low Ly-6G + γIMCs in splenocytes from mice infected with NIH34, were isolated by FACS. ( b , c ) Cytospin preparations of each sorted cell type were visualized with May-Grünwald-Giemsa staining ( b ), whereas intracellular IFN-γ (green, IFN-γ; red, nuclei) was visualized with a confocal laser microscopy ( c ). Scale bars, 20 μm. ( d , e ) Paraffin-embedded sections of peritoneum, from mice i.p. infected with NIH34 and skin from mice subcutaneously (s.c.) infected with NIH34 for 48 h ( d ), and of spleen and kidney from mice i.p. infected with or without K33 or NIH34 for 48 h, ( e ) were visualized with hematoxylin and eosin staining. The yellow arrows indicate the cells with ring-shaped nuclei. Scale bars, 100 μm. ( f ) Sorted IMCs were cultured with control medium (Med), G-CSF (50 ng ml −1 ), M-CSF (10 ng ml −1 ), GM-CSF (10 ng ml −1 ), or IL-5 (10 ng ml −1 ) for 2–4 days, and their absolute numbers were counted on the indicated days. Data are expressed as the average (mean±s.d.) of triplicate wells ( n =3). The differences compared with Med were statistically significant (** P <0.01) as determined by Student's t -test. ( g ) γIMCs (blue line) and GM-CSF (2 days)-cultured γIMCs (GM2-γIMCs: red line) were stained for the indicated markers. Data are representative of three independent experiments. ( h ) Cytospin preparations of GM2-γIMCs were visualized with May-Grünwald-Giemsa staining. Scale bars, 20 μm. ( i , j ) γIMCs and GM2-γIMCs were cultured with erythromycin-treated NIH34 (MOI 100) in the presence of control rat IgG or an IFN-γ neutralizing mAb (clone R4-6A2) for 24 h. The levels of IFN-γ ( i ) and NO 2 − ( j ) in the culture supernatants were measured by ELISA and Griess reagent system, respectively. The average (mean±s.d.) of triplicate wells is shown. Statistical significance (** P <0.01) was determined by ANOVA. Full size image Nitric oxide (NO) is considered to be a main mechanism for controlling some infective agents. Myeloid cells are able to release NO in response to IFN-γ [30] , [31] , [32] , [33] ; moreover, IFN-γ and NO-producing myeloid cells have been described in cancer [34] . Therefore, we investigated the ability of γIMCs to produce NO in response to GAS. When stimulated by autocrine and/or paracrine IFN-γ, γIMCs (but not than PMNs and granulocyte-like cells differentiated from γIMCs using GM-CSF) were able to produce NO, because their NO production was significantly blocked in the presence of IFN-γ neutralizing mAb ( Fig. 5j ). Differentiation of precursor-like cells into γIMCs Bone marrow contains the highest proportion of γIMCs ( Fig. 4c and d ). Therefore, we attempted to identify the precursors of γIMCs in the bone marrow of mice infected with severe invasive GAS isolates. Interestingly, analysis of the surface molecules revealed 2 distinct subsets of IFN-γ-producing cells ( Fig. 6a ): a minor and a major subset. The minor subset constituted 6.9±3.2% of IFN-γ-producing bone marrow cells ( Fig. 6b ), and comprised CD11b + CD11c − F4/80 low Ly-6G + large cells ( Supplementary Fig. S6 ), containing ring-shaped nuclei (BM-γIMCs) ( Fig. 6c ). On the basis of morphology and surface phenotype, these cells corresponded to splenic γIMCs (Sp-γIMCs) ( Fig. 5a and b ). Neither isolated BM-γIMCs nor Sp-γIMCs proliferated in the presence of GM-CSF ( Figs 5f and 6d ). These cells differed from metamyelocytes and immature neutrophils in non-infected bone marrow ( Fig. 6c ). The major subset of IFN-γ-producing cells comprised CD11b + CD11c low F4/80 + Ly-6G low precursor-like cells (BMPCs) ( Fig. 6b ; Supplementary Fig. S6 ), which constituted 74.8±13.7% of IFN-γ-producing cells ( Fig. 6b ). This subset consisted of ∼ 10% monocyte-like ring cells and immature myeloid cells ( Fig. 6c ), which are phenotypically different from CD11b − Ly-6G − cells such as granulocyte–monocyte progenitors, common myeloid progenitors, and myelolymphoid progenitors [35] . In the presence of GM-CSF, isolated BMPCs proliferated ( Fig. 6d ) and differentiated into BM-γIMCs ( Fig. 6c and e ). Moreover, after 2 extra days of incubation with GM-CSF, differentiated BM-γIMCs increased their expression of CD11c, F4/80, DX5 and Siglec-F ( Fig. 6f ). The polymorphonuclear and cell surface phenotype ( Supplementary Fig. S6 ) was similar to that of Sp-γIMCs cultured with GM-CSF ( Fig. 5g and h ). The differentiation of BMPCs into BM-γIMCs was totally blocked in the presence of IFN-γ neutralizing mAb; by contrast, this cytokine was dispensable for differentiation into granulocyte-like cells ( Supplementary Fig. S6 ). These results are in accordance with the absence of Ly-6G + γIMCs in the spleen of GAS-infected C57BL6. Ifng −/− mice ( Supplementary Fig. S7 ). The expression level of Ly-6G in PMNs was similar for WT and Ifng −/− mice ( Supplementary Fig. S7 ). As with γIMCs and γIMC-differentiated granulocyte-like cells ( Fig. 5i ), the cells differentiated from BMPCs, after 2 extra days of incubation with GM-CSF, retained the ability to release IFN-γ in response to GAS; however, subsequent differentiation by GM-CSF reduced the ability to produce IFN-γ ( Fig. 6g ). A few IFN-γ-producing cells in non-infected mice were recognized in the same fraction as the BMPCs ( Fig. 6a ), and, therefore, it is possible that BMPCs exist in the naïve bone marrow. Our results suggest that IFN-γ-producing BMPCs are the precursors of γIMCs, and that their differentiation is dependent on autocrine and/or paracrine pathways involving IFN-γ. Notably, the BMPC-derived unclassified granulocyte-lineage, such as γIMCs (but not immature PMNs), seems to appear during severe invasive GAS infections. 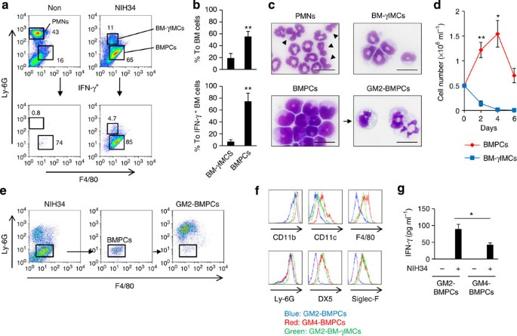Figure 6: BMPCs differentiate into γIMCs in the presence of GM-CSF. (a) C3H/HeN mice non-infected or i.p. infected with NIH34 (3.0×107CFU per mouse) for 42 h were i.v. injected with monensin. Six hours later, the mice were killed and their bone marrow cells were immediately stained for the indicated markers, and analysed by ICS assay. Lower panels show the cells gated on the IFN-γ+population. The numbers (%) in the plots represent the proportion of PMNs, BM-γIMCs, and BMPCs to total (upper panels) and IFN-γ+(lower panels) bone marrow cells. (b) Proportion (%) of BM-γIMCs and BMPCs to bone marrow cells (upper panel) or IFN-γ-producing bone marrow cells (lower panel). Data are expressed as mean±s.d. (n=3). The differences compared with the proportion of BM-γIMCs were statistically significant (**P<0.01) as determined by Student'st-test. (c) Cytospin preparations of sorted PMNs, BM-γIMCs, BMPCs, and GM-CSF (2 days)-cultured BMPCs (GM2-BMPCs) were visualized with May-Grünwald-Giemsa staining. Arrowheads indicate stab neutrophils or metamyelocytes. Scale bars, 20 μm. (d) Sorted BMPCs and BM-γIMCs were cultured with GM-CSF (10 ng ml−1) for 2–6 days, and their absolute numbers were counted on the indicated days. Data are expressed as mean±s.d. (n=3). The differences in proliferation increase were statistically significant (*P<0.05, **P<0.01) as determined by Student'st-test. (e) Flow cytometry profile of infected bone marrow cells (left), sorted BMPCs (middle), and GM2-BMPCs (right). Rectangles show a sorting gate of BMPCs. (f) GM-CSF-cultured BMPCs (2 days or 4 days; GM2-BMPCs, blue line; GM4-BMPCs, red line) and BM-γIMCs (2 days; GM2-BM-γIMCs, green line) were stained for the indicated markers. Data are representative of 3 independent experiments. (g) IFN-γ production from BMPCs. GM2-BMPCs or GM4-BMPCs were cultured with erythromycin-treated NIH34 (MOI 100) in the presence of control rat IgG or an IFN-γ neutralizing mAb (clone R4-6A2) for 24 h. The level of IFN-γ in the culture supernatants was measured by ELISA. The average (mean±s.d.) of triplicate wells is shown. Statistical significance (*P<0.05) was determined by Student'st-test. Figure 6: BMPCs differentiate into γIMCs in the presence of GM-CSF. ( a ) C3H/HeN mice non-infected or i.p. infected with NIH34 (3.0×10 7 CFU per mouse) for 42 h were i.v. injected with monensin. Six hours later, the mice were killed and their bone marrow cells were immediately stained for the indicated markers, and analysed by ICS assay. Lower panels show the cells gated on the IFN-γ + population. The numbers (%) in the plots represent the proportion of PMNs, BM-γIMCs, and BMPCs to total (upper panels) and IFN-γ + (lower panels) bone marrow cells. ( b ) Proportion (%) of BM-γIMCs and BMPCs to bone marrow cells (upper panel) or IFN-γ-producing bone marrow cells (lower panel). Data are expressed as mean±s.d. ( n =3). The differences compared with the proportion of BM-γIMCs were statistically significant (** P <0.01) as determined by Student's t -test. ( c ) Cytospin preparations of sorted PMNs, BM-γIMCs, BMPCs, and GM-CSF (2 days)-cultured BMPCs (GM2-BMPCs) were visualized with May-Grünwald-Giemsa staining. Arrowheads indicate stab neutrophils or metamyelocytes. Scale bars, 20 μm. ( d ) Sorted BMPCs and BM-γIMCs were cultured with GM-CSF (10 ng ml −1 ) for 2–6 days, and their absolute numbers were counted on the indicated days. Data are expressed as mean±s.d. ( n =3). The differences in proliferation increase were statistically significant (* P <0.05, ** P <0.01) as determined by Student's t -test. ( e ) Flow cytometry profile of infected bone marrow cells (left), sorted BMPCs (middle), and GM2-BMPCs (right). Rectangles show a sorting gate of BMPCs. ( f ) GM-CSF-cultured BMPCs (2 days or 4 days; GM2-BMPCs, blue line; GM4-BMPCs, red line) and BM-γIMCs (2 days; GM2-BM-γIMCs, green line) were stained for the indicated markers. Data are representative of 3 independent experiments. ( g ) IFN-γ production from BMPCs. GM2-BMPCs or GM4-BMPCs were cultured with erythromycin-treated NIH34 (MOI 100) in the presence of control rat IgG or an IFN-γ neutralizing mAb (clone R4-6A2) for 24 h. The level of IFN-γ in the culture supernatants was measured by ELISA. The average (mean±s.d.) of triplicate wells is shown. Statistical significance (* P <0.05) was determined by Student's t -test. Full size image Distinction between γIMCs and MDSCs MDSCs are composed of F4/80 − or F4/80 low granulocytic MDSCs with ring-shaped nuclei, and F4/80 + monocytic MDSCs [10] , [11] . They can produce IFN-γ [13] . Furthermore, granulocytic/monocytic MDSCs differentiate into CD11c + F4/80 + Gr-1 + cells [12] , as do γIMCs ( Fig. 5g ). To identify the relationship between the types of γIMCs observed during severe invasive GAS infections and MDSCs, we investigated the ability of γIMCs to suppress T-cell responses. As reported previously, in vitro -differentiated Ly-6C + Ly-6G low F4/80 + MDSCs [9] spontaneously produced IFN-γ ( Fig. 7a ), and inhibited Ag-specific T-cell proliferation and IFN-γ production from T cells ( Fig. 7b ). Conversely, purified γIMCs failed to inhibit T-cell responses ( Fig. 7c ), suggesting that γIMCs are functionally distinct from MDSCs. Additionally, MDSCs markedly decreased in number and lost the ability to produce IFN-γ when cultured in vitro with severe invasive GAS isolates ( Fig. 7a ). Furthermore, CCR2 − CX3CR1 + CD31 + γIMCs are phenotypically different from CCR2 + CX3CR1 − CD31 − granulocytic MDSCs and CCR2 high CX3CR1 − CD31 + monocytic MDSCs ( Supplementary Table S1 ). Taken together, our results indicate that γIMCs, which appear in association with severe invasive GAS infections, comprise a novel subset of IFN-γ-producing cells, but not MDSCs. 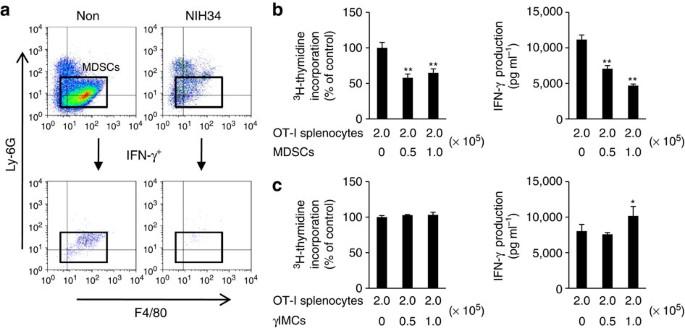Figure 7: γIMCs are functionally different from MDSCs. (a) C57BL/6 mouse bone marrow-derived MDSCs were differentiatedin vitrowith 40 ng ml−1GM-CSF for 4 days. MDSCs were then incubated with or without severe invasive GAS isolates (NIH34; MOI 1) in the presence of brefeldin A (10 μg ml−1). Three hours later, the cells were immediately stained for F4/80, Ly-6G, and IFN-γ, and analysed by ICS assay. Lower panels show the cells gated on the IFN-γ+population. (b,c) CD11b+CD11c−Ly-6C+Ly-6Glowin vitro-differentiated MDSCs, and CD11b+CD11c−F4/80lowLy-6G+γIMCs, in the spleen from C57BL per six mice infected with NIH34 (3.0×107CFU per mouse) for 48 h were isolated by FACS. Purified MDSCs (b) or purified γIMCs (c) were cultured at the indicated ratio with 2.0×105splenocytes from C57BL/6.OT-I mice in the presence of antigenic OVA357–364peptides. Cell proliferation was measured using [3H] thymidine uptake, and the level of IFN-γ in the culture supernatants was measured by ELISA. Each experiment was performed in triplicate. Mean±s.d. is shown. The differences compared with OT-I splenocytes alone were statistically significant (*P<0.05, **P<0.01) as determined by ANOVA. Data are representative of three independent experiments. Figure 7: γIMCs are functionally different from MDSCs. (a) C57BL/6 mouse bone marrow-derived MDSCs were differentiated in vitro with 40 ng ml −1 GM-CSF for 4 days. MDSCs were then incubated with or without severe invasive GAS isolates (NIH34; MOI 1) in the presence of brefeldin A (10 μg ml −1 ). Three hours later, the cells were immediately stained for F4/80, Ly-6G, and IFN-γ, and analysed by ICS assay. Lower panels show the cells gated on the IFN-γ + population. ( b , c ) CD11b + CD11c − Ly-6C + Ly-6G low in vitro -differentiated MDSCs, and CD11b + CD11c − F4/80 low Ly-6G + γIMCs, in the spleen from C57BL per six mice infected with NIH34 (3.0×10 7 CFU per mouse) for 48 h were isolated by FACS. Purified MDSCs ( b ) or purified γIMCs ( c ) were cultured at the indicated ratio with 2.0×10 5 splenocytes from C57BL/6.OT-I mice in the presence of antigenic OVA 357–364 peptides. Cell proliferation was measured using [ 3 H] thymidine uptake, and the level of IFN-γ in the culture supernatants was measured by ELISA. Each experiment was performed in triplicate. Mean±s.d. is shown. The differences compared with OT-I splenocytes alone were statistically significant (* P <0.05, ** P <0.01) as determined by ANOVA. Data are representative of three independent experiments. Full size image Role of γIMCs in severe invasive GAS infections To elucidate the protective role of γIMCs, we employed an adoptive transfer system using WT or Ifng −/− mice. CD11b + CD11c − F4/80 low Ly-6G + γIMCs were purified from the spleens of WT mice infected with severe invasive GAS at day 2, and transferred into recipient mice. These mice were infected with a lethal dose of severe invasive GAS isolates (5×10 7 CFU (high dose)/WT mouse, 1×10 7 CFU (low dose)/ Ifng −/− mouse), and the bacterial loads (CFUs) in the blood were quantified. At 24 h post-infection, γIMC-recipients and IFN-γ-treated mice had significantly lower bacterial loads in the blood than did control mice ( Fig. 8a–c ). Additionally, all control mice and all IFN-γ-treated mice died. By contrast, 100% of high dose-infected WT recipients and low dose-infected Ifng −/− recipients of γIMCs, and also low dose-infected WT mice, survived until 60 h post-infection ( Fig. 8d–f ). Our results indicate that IFN-γ successfully improved the bacterial clearance, but that systemic IFN-γ treatment was detrimental to survival following GAS infections ( Fig. 8a,c,d and f ). Thus, it appears that γIMCs have a protective role in severe invasive GAS infections. 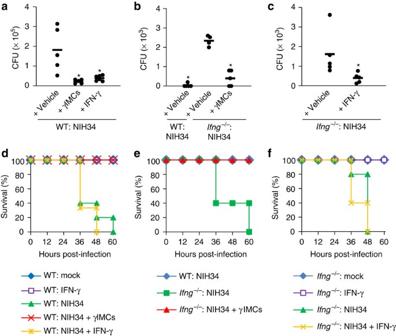Figure 8: γIMCs participate in protection against severe invasive GAS infections. (a–f) CD11b+CD11c−F4/80lowLy-6G+γIMCs in the spleen from C57BL/6 WT mice infected with NIH34 (3.0×107CFU per mouse) for 48 h were isolated by FACS. WT orIfng−/−mice i.v. received 3.0×106γIMCs, or were i.p. treated with IFN-γ (10 ng per mouse). (a,d) WT mice (n=5), WT recipients of γIMCs (n=5), and mice i.p. treated with IFN-γ (n=6) were i.p. inoculated with NIH34 (5.0×107CFU per mouse). (b,e) WT mice (n=5),Ifng−/−mice (n=5), andIfng−/−recipients of γIMCs (n=5) were i.p. inoculated with NIH34 (1.0×107CFU per mouse). (c,f)Ifng−/−mice (n=5) andIfng−/−mice i.p. treated with IFN-γ (n=5) were i.p. inoculated with NIH34 (1.0×107CFU per mouse). (a,b,c) The CFU of NIH34 in the peripheral blood was determined at 24 h post-infection. The differences compared with NIH34-infected WT mice (a) or NIH34-infectedIfng−/−mice (b,c) were statistically significant (*P<0.05) as determined by the Mann–WhitneyU-test. (d,e,f) Survival was observed for 60 h post-infection. Data are representative of two independent experiments. Figure 8: γIMCs participate in protection against severe invasive GAS infections. ( a – f ) CD11b + CD11c − F4/80 low Ly-6G + γIMCs in the spleen from C57BL/6 WT mice infected with NIH34 (3.0×10 7 CFU per mouse) for 48 h were isolated by FACS. WT or Ifng −/− mice i.v. received 3.0×10 6 γIMCs, or were i.p. treated with IFN-γ (10 ng per mouse). ( a , d ) WT mice ( n =5), WT recipients of γIMCs ( n =5), and mice i.p. treated with IFN-γ ( n =6) were i.p. inoculated with NIH34 (5.0×10 7 CFU per mouse). ( b , e ) WT mice ( n =5), Ifng −/− mice ( n =5), and Ifng −/− recipients of γIMCs ( n =5) were i.p. inoculated with NIH34 (1.0×10 7 CFU per mouse). ( c , f ) Ifng −/− mice ( n =5) and Ifng −/− mice i.p. treated with IFN-γ ( n =5) were i.p. inoculated with NIH34 (1.0×10 7 CFU per mouse). ( a , b , c ) The CFU of NIH34 in the peripheral blood was determined at 24 h post-infection. The differences compared with NIH34-infected WT mice ( a ) or NIH34-infected Ifng −/− mice ( b , c ) were statistically significant (* P <0.05) as determined by the Mann–Whitney U -test. ( d , e , f ) Survival was observed for 60 h post-infection. Data are representative of two independent experiments. Full size image Previous studies have indicated that T cells and NK cells may have a role in the production of IFN-γ during GAS infections [5] , [15] , [16] , [17] , [19] , [20] , [21] . In the present study, we have demonstrated for the first time that γIMCs in the peritoneal cavity, skin, spleen, kidney, peripheral blood and bone marrow (but not T cells or NK cells) produce IFN-γ in vivo during the early stage of severe invasive GAS infections. The intensity of IFN-γ production is comparable among γIMCs, T cells, and NK cells, but production by γIMCs takes place sooner than that by T cells and NK cells. Moreover, throughout the course of GAS infection, γIMCs are the main IFN-γ-producing cells in the spleen. We further observed that IFN-γ neutralized Rag −/− mice succumbed to severe GAS infection at a similar rate to WT mice. Taken together, our results indicate that γIMCs comprise the major source of IFN-γ during the early stage of severe invasive GAS infections, and that they have an important protective role. Notably, IFN-γ administration reduced the number of bacteria in the blood, whereas the transfer of γIMCs, but not of IFN-γ, improved the survival rate of mice following GAS infection. Therefore, IFN-γ was necessary, but not sufficient, to protect mice from severe invasive GAS infections. We propose that NO production from γIMCs (which is restrictively controlled by IFN-γ), perhaps combined with that from other myeloid cells, may have a critical defensive role during the early stage of infection. In systemic GAS infection, γIMCs are deployed in various infected tissues; thus, the derived IFN-γ, NO, and/or as yet unidentified protective factors may promote the development of innate immune responses for the activation of phagocytes. However, we were unable to exclude the possibility that excessive quantities of IFN-γ secreted by T cells following superantigens stimulation, by NK cells, and even by γIMCs at the late stage of infection, are detrimental to survival following GAS infections, by exacerbating inflammatory responses and organ injury. γIMCs express phenotypic markers of the monocyte/macrophage and granulocyte lineages, and are phenotypically different from other Ly-6C + cells, such as inflammatory and resident monocytes [11] , [36] . Mature PMNs, immature PMNs, and their progenitors proliferate or maintain their survival in the presence of G-CSF [37] . By contrast, in the present study, γIMCs did not survive in the presence of G-CSF. However, in the presence of GM-CSF, they differentiated into a PMN-like phenotype. Thus, γIMCs are distinct from the PMN lineage that develops during steady-state haematopoiesis. In the presence of GM-CSF, γIMCs possessed the ability to express a specific marker for Eos, Siglec-F. Nevertheless, based on staining with H7 and T21, they were distinct from Siglec-F + splenic Eos. Our observation that γIMCs failed to proliferate in response to IL-5 are consistent with the previous finding that T21 mAb may recognize IL-5Rα and other myeloid cell surface protein(s) [38] . Thus, γIMCs are unlikely to be committed to an Eos lineage; similarly, they are phenotypically different from DX5 + basophils and basophil lineage-committed progenitors [39] . Granulocytic MDSCs are very similar to γIMCs in terms of surface markers (CD11b, F4/80, Ly-6C, Ly-6G, CD44, CD49d, and CD62L) [10] , [11] , dependency on a growth factor (GM-CSF) [12] , and cytokine production profile (IFN-γ) [13] . However, in the present study, we reveal that MDSCs did not produce IFN-γ in response to in vitro GAS infections. This is consistent with the previous finding that MDSCs from septic mice did not produce IFN-γ [40] . MDSCs are believed to originate from, or be accelerated by, the blockade of normal haematopoiesis during chronic inflammation or in a tumour-bearing state. γIMCs and MDSCs may therefore be closely related cell populations, and their differentiation and function may be regulated by the host circumstances. On the basis of our present findings, we conclude that γIMCs are committed to an unclassified granulocyte lineage with an immature phenotype, and that such cells have the potential to replenish granulocyte populations. Moreover, GM-CSF is essential for the extraordinary state, such as severe systemic infection, but not for normal haematopoiesis [41] . The replacement of GM-CSF-dependent γIMCs may be regarded as a marked shift to the left of the leukocyte differential, with many immature granulocytes in automated cell counting. This is a characteristic of severe invasive GAS infections in our mouse model and also in human diseases [4] , [28] . The role of γIMCs in other infections and inflammatory diseases remains to be elucidated. In the present study, we reveal that γIMCs differentiate from a subpopulation of CD11b + CD11c low F4/80 + Ly-6G low cells in the bone marrow; this is known as a monocyte lineage. No γIMCs were detected in Ifng −/− mice infected with GAS, and IFN-γ-producing BMPCs (but not γIMCs) failed to differentiate into granulocyte-like cells in the presence of an IFN-γ neutralizing mAb. These observations suggest that the generation of γIMCs depends on the production of IFN-γ by BMPCs themselves. IFN-γ derived from BMPCs and γIMCs may be a key component of haematopoiesis during innate and adaptive immune responses, as shown in cases of malaria and Mycobacterium avium infection [35] , [42] . In the steady state, a few IFN-γ-producing cells existed in the Ly-6C low CD31 + fraction, including mixed progenitors of bone marrow [43] . Thus, we cannot exclude the possibility that BMPCs exist in non-infected bone marrow and have potential to produce IFN-γ, and that a subset of bone marrow cells can produce IFN-γ for the reproduction of haematopoietic stem cells [42] . Ring cells are present in the blood and bone marrow of humans, especially patients with chronic myeloproliferative diseases [6] , [7] , [8] but only rarely in healthy control subjects [7] . Further investigations of peripheral blood leukocytes or bone marrow cells from severe invasive GAS patients are required, to clarify whether the human counterpart of γIMCs is a major source of IFN-γ in STSS patients. PMNs are known to be essential for protection against non-invasive streptococcal infections. Following infection with severe invasive strains, PMNs are impaired by enhanced virulence factors (for example, streptolysin O) [18] , [27] , and therefore other protective mechanisms are required for the recovery. The results of our present study indicate that γIMCs, a novel class of differentiated granulocytic ring cells, which comprise the major source of IFN-γ during the early phase of severe invasive GAS infections, may have an important role. During the later stage of infection, IFN-γ derived from T cells and NK cells may be detrimental to the host. Nevertheless, we believe that the orchestrated regulation of γIMCs serves as a protective mechanism against severe invasive bacterial infections. Bacterial strains The STSS criteria in this study are based on those proposed by the Working Group on Severe Streptococcal Infections [44] . The clinical isolates from STSS (NIH34 ( emm3 genotype], NIH230 ( emm49 genotype), NIH186 ( emm1 genotype), and NIH202-2 ( emm1 genotype)), and also from non-invasive infections (K33 ( emm3 genotype)), were collected by the Working Group for Beta-hemolytic Streptococci in Japan [18] , [27] . Mice All work performed using mice was carried out in accordance with the guidelines for animal care approved by National Institute of Infectious Diseases. C3H/HeN and C57BL/6 mice (male, 5–6-weeks-old) were purchased from SLC. C57BL/6. Rag1−/− (ref. 26 ) and C57BL/6. Ifng−/− (ref. 45 ) mice were purchased from the Jackson Laboratory. All mice were maintained in a specific pathogen-free condition. GAS infections in a mouse model GAS were grown to late-log phase (OD 600 =0.75–0.95). Then, 1.0×10 7 CFU to 5.0×10 7 CFU GAS, suspended in 0.5 ml PBS, were i.p. inoculated into 6–8-week-old male mice. In some experiments, mice were i.p. administered with 1 mg of an anti-mouse IFN-γ neutralizing mAb (clone R4-6A2) or control rat IgG, or 10 ng of recombinant mouse IFN-γ (Wako Pure Chemical Industries) at infection. Plasma production of CXCL10 (an IFN-γ-inducible protein) at 24 h, after NIH34 infection, was used to assess the activity of inoculated IFN-γ (10 ng per mouse) in Ifng −/− recipients ( Ifng −/− mice, 230.1±58.2 pg ml −1 ; IFN-γ-treated Ifng −/− mice, 468.2±147.2 pg ml −1 *; C57BL/6 mice as positive control, 460.6±126.9 pg ml −1 *). Data were expressed as mean±s.d. ( n =5). The differences compared with Ifng −/− mice were statistically significant (* P <0.05) as determined by Student's t -test. Survival curves were compared using a log-rank test. Measurement of cytokines in plasma The plasma cytokine levels were determined by FlowCytomix (eBioscience) using a FACSCalibur flow cytometer (Becton, Dickinson and Company (BD)), according to the manufacturer's instructions. Flow cytometry analysis For the in vivo ICS assay [22] , [23] , at day 2 post-infection, mice were intravenously (i.v.) injected with 500 μl of a PBS solution containing 100 μg monensin (Sigma-Aldrich) at 6 h before collecting. Splenocytes, peripheral blood cells, bone marrow cells, and leukocytes in the peritoneal cavity, kidney, and skin were collected and rapidly processed on ice. Single-cell suspensions were prepared, and red blood cells were removed using an ammonium chloride lysis buffer. For the in vitro ICS assay, non-infected or infected cells were cultured with 10 μg ml −1 brefeldin A (Sigma-Aldrich) for 3 h. One million cells were stained with Alexa Fluor 488-, FITC-, PE-, Alexa Fluor 647-, allophycocyanin (APC)-, or Pacific Blue-conjugated Abs (clones and suppliers, Supplementary Table S2 ) at 4 °C for 15 min. Nonspecific staining was blocked with an anti-mouse FcγR mAb (clone 2.4G2). Dead cells were excluded by 7-aminoactinomycin D (7-AAD; Sigma-Aldrich) staining. After washing, cells were fixed in 2% paraformaldehyde/PBS for 10 min and then permeabilized in 0.5% saponin/0.5% BSA/PBS (permeabilization buffer), before being stained with a PE- or APC-conjugated anti-mouse IFN-γ mAb (clone XMG1.2; eBioscience) or isotype control Ab (eBioscience) for 45 min at 4 °C. Cells were washed, first with permeabilization buffer, then with FACS buffer, before being applied to a FACSCalibur or FACSAria flow cytometer (BD). Analyses were performed using FlowJo software (Ashland, OR). Cytological analysis Fifty thousand cells were subjected to a cytospin (Thermo Shandon). For morphological analysis, the cytospin preparations were fixed with methanol and visualized with May-Grünwald-Giemsa staining. For intracellular IFN-γ staining, the cytospin preparations were fixed with 2% paraformaldehyde for 10 min, treated with 50 m M NH 4 Cl/PBS for 15 min, and blocked with an anti-mouse FcγR mAb (clone 2.4G2) in permeabilization buffer for 15 min. Slides were stained with an APC-conjugated anti-mouse IFN-γ mAb (clone XMG1.2) or isotype control Ab (eBioscience) for 45 min, washed 3 times with permeabilization buffer, and then washed 3 times with PBS. Nuclei were visualized with propidium iodide staining. Samples were viewed and photographed with a Carl Zeiss LSM510 confocal laser scanning microscope. Histology For histological analysis, the tissues from GAS-infected mice were fixed in 10% formalin/PBS. The paraffin-embedded sections were stained with hematoxylin and eosin. In vitro culture of γIMCs and BMPCs Purified CD11b + CD11c − F4/80 low Ly-6G + γIMCs and CD11b + CD11c low F4/80 + Ly-6G low BMPCs from GAS-infected (monensin-untreated) mice were cultured at 0.5×10 6 cells per ml in medium containing RPMI 1640 (Wako) with 10% FBS (Nichirei), 100 U ml −1 penicillin, 10 μg ml −1 streptomycin, 2 mM glutamine, 25 mM HEPES, and 50 μM 2-ME, with or without 10–50 ng ml −1 recombinant mouse GM-CSF, G-CSF, M-CSF, or IL-5 (R&D Systems), in the presence or absence of 1 μg ml −1 control rat IgG or R4-6A2, for 2–6 days. On days 2 and 4, 50% of the medium was replaced with fresh medium, or the cells were collected for May-Grünwald-Giemsa staining and flow cytometry analysis. In some experiments, the cells were cultured at 0.5×10 6 cells ml −1 with 25 μg ml −1 erythromycin and NIH34 (MOI 100) in 10% FBS/phenol red-free RPMI medium, supplemented with 10 ng ml −1 GM-CSF, in the presence of 1 μg ml −1 control rat IgG or R4-6A2 for 24 h. The levels of IFN-γ and NO in the culture supernatants were measured by an instant ELISA kit (eBioscience) and a Griess reagent (Wako), respectively, according to the manufacturer's instructions. In vitro culture of Eos and MDSCs For obtaining Eos, naïve bone marrow cells were cultured in 10% FBS/RPMI medium supplemented with stem cell factor (PeproTech) and FLT3-ligand (PeproTech) for 4 days, and then with medium containing recombinant mouse IL-5 (R&D Systems). On day 12, the cells were collected for May-Grünwald-Giemsa staining and flow cytometry analysis [46] . To isolate bone marrow-derived MDSCs, naïve bone marrow cells were cultured at 1.0×10 6 cells per ml in 10% FBS/RPMI medium, supplemented with 40 ng ml −1 GM-CSF. On day 4, the cells were collected for FACS analysis of CD11b + CD11c − Ly-6C + Ly-6G low MDSCs [9] . Ag-specific T-cell proliferation and IFN-γ production The Ag-specific proliferation of CD8 + T cells was evaluated using OT-I OVA-specific MHC Class I-restricted TCR transgenic mice. Varying amounts of purified CD11b + CD11c − F4/80 low Ly-6G + γIMCs from infected C57BL/6 mice at 2 days post-infection, or bone marrow-derived F4/80 + Ly-6C + Ly-6G low MDSCs, were added to 2.0×10 5 naïve splenocytes from OT-I mice in medium containing RPMI 1640 with 10% FBS in a U-bottom 96-well plate. These co-cultures were stimulated with antigenic OVA 357–364 peptides (10 μM) for 4 days. Proliferation of OT-I cells in triplicate was estimated by the incorporation of [ 3 H] thymidine (1 μCi (0.0037 MBq) per well), added at 18 h before cell harvest. The level of IFN-γ in the culture supernatants was measured by an instant ELISA kit (eBioscience), according to the manufacturer's instructions. Adoptive transfer of γIMCs CD11b + CD11c − F4/80 low Ly-6G + γIMCs in splenocytes from Ifng +/+ mice infected with NIH34 (3.0×10 7 CFU) for 48 h were isolated with a FACSAria flow cytometer. Recipient mice were i.v. administered with purified CD11b + CD11c − F4/80 low Ly-6G + γIMCs (3.0×10 6 cells), and i.p. inoculated with NIH34 (1.0×10 7 CFU to 5.0×10 7 CFU) on the same day. Measurement of bacterial loads At 24 h post-infection, 20 μl of peripheral blood was removed from the tail vein by phlebotomy. The blood was diluted at 1:10–1:1000 with PBS and spread on a Columbia agar plate containing 5% sheep blood (BD). To determine the number of NIH34 in peripheral blood, the plates were incubated for 20 h at 37 °C in a 5% CO 2 atmosphere, and the colonies were counted. The number of NIH34 was compared statistically using the Mann–Whitney U -test. How to cite this article: Matsumura, T. et al . Interferon-γ-producing immature myeloid cells confer protection against severe invasive group A Streptococcus infections Nat. Commun. 3:678 doi: 10.1038/ncomms1677 (2012).